Mouse and human strategies identifyPTPN14as a modifier of angiogenesis and hereditary haemorrhagic telangiectasia Hereditary haemorrhagic telangiectasia (HTT) is a vascular dysplasia syndrome caused by mutations in transforming growth factor-β/bone morphogenetic protein pathway genes, ENG and ACVRL1. HTT shows considerable variation in clinical manifestations, suggesting environmental and/or genetic modifier effects. Strain-specific penetrance of the vascular phenotypes of Eng +/− and Tgfb1 −/− mice provides further support for genetic modification of transforming growth factor-β pathway deficits. We previously identified variant genomic loci, including Tgfbm2 , which suppress prenatal vascular lethality of Tgfb1 −/− mice. Here we show that human polymorphic variants of PTPN14 within the orthologous TGFBM2 locus influence clinical severity of HTT, as assessed by development of pulmonary arteriovenous malformation. We also show that PTPN14 , ACVRL1 and EFNB2 , encoding EphrinB2, show interdependent expression in primary arterial endothelial cells in vitro. This suggests an involvement of PTPN14 in angiogenesis and/or arteriovenous fate, acting via EphrinB2 and ACVRL1/activin receptor-like kinase 1. These findings contribute to a deeper understanding of the molecular pathology of HTT in particular and to angiogenesis in general. The transforming growth factor (TGF)-β signalling pathway is critical in many common diseases, including fibrosis, cancer, cardiovascular and autoimmune disorders [1] . TGF-β and BMP (bone morphogenetic protein) signalling pathways are also disrupted in single gene disorders, including Loeys–Dietz syndrome [2] , thoracic ascending aortic dissections [3] , multiple self-healing squamous epithelioma [4] , Marfan syndrome [3] , juvenille polyposis syndrome [5] , familial pulmonary hypertension [6] and hereditary haemorrhagic telangiectasia (HHT) [7] , [8] , with a notable theme of the TGF-β spectrum disorders being variable expressivity of clinical features [9] . HHT is one of the most common monogenic diseases. It is autosomal dominant, affects at least 1 in 5,000 individuals worldwide and is under-reported due to clinical unfamiliarity with the disease [7] , [8] . It is a multivisceral vascular disease with incomplete, age-dependent penetrance of clinical features, caused predominantly by mutations in the genes ENG (HHT1) or ACVRL1 (HHT2). The encoded proteins, endoglin and activin receptor-like kinase 1 (ALK1), respectively, are endothelial receptors involved in TGF-β superfamily signalling [10] , [11] . HHT patients typically present during adolescence with recurrent nosebleeds or epistaxis, and with cutaneous telangiectases, which are clusters of abnormally dilated vessels caused by defective vascular remodelling and capillary breakdown [7] , [12] . These manifestations are highly penetrant (85%) but show variable expressivity [13] . More serious visceral complications of HHT are caused by larger arteriovenous malformations (AVMs) that include pulmonary (PAVM), hepatic and cerebral AVMs, as well as gastrointestinal bleeding from mucosal telangiectases that can cause severe anemia [14] . Globally, PAVM is found in ∼ 50% of HHT patients and causes right-to-left shunting, because the pulmonary capillary filter is compromised. This allows clots to enter the systemic circulation, that can lead to frequent severe complications, often at a young age, including stroke, transient ischaemic attack and brain abscess [15] . Massive haemoptysis and bleeding into the pleural cavity is less common. Screening for PAVMs is therefore recommended to HHT patients and their asymptomatic relatives. Genotype–phenotype correlation studies have shown that the prevalence of PAVM is significantly higher in HHT1 than in HHT2 (refs 13 , 16 ). There are also differences in the prevalence of PAVM in HHT that are at least partially attributable to population-specific variations in the HHT1:HHT2 ratio [17] . In France and Italy, HHT2 is more common than HHT1, with consequent lower incidence of PAVM. In the Netherlands, HHT1 is the most common form [13] , and in the Dutch Antilles, all cases of HHT are HHT1 (ref. 18 ). Thus, PAVM is of higher incidence in Dutch versus Franco–Italian populations. There has been debate as to whether HHT is a disorder of TGF-β or BMP signalling. This superfamily contains over 30 related ligands, including TGF-βs, BMPs, growth/differentiation factors and activins. The major ligand sub-classes possess distinct and specific type II serine–threonine receptor kinases, but type I receptor kinases are promiscuous, can hetero-oligomerize with a variety of type II and I receptors, and are activated by a broader range of superfamily ligands [1] . TGF-βs generally signal via the canonical TβRII, TβRI, Smad2/Smad3/Smad4 pathway and BMPs through BMPR2, BMPR1A and/or BMPR1B via Smad1/Smad5/Smad8. Biochemically, ALK1 was first designated as a TGF-β type 1 serine–threonine receptor kinase [19] , and endoglin as a type III TGF-β co-receptor [20] . However, endoglin can bind a variety of other superfamily ligands, including BMPs and activin [21] , and the ligand with highest affinity for ALK1 is BMP9 (ref. 22 , which triggers signalling via the canonical Smad1/Smad5/Smad8 pathway, therefore implicating HHT as a 'BMP disease'. Conversely, mouse genetics studies implicate functional interaction between the bona fida TGF-β pathway and endoglin/ALK1. Specifically, Acvrl1 −/− and Eng −/− embryos manifest prenatal-lethal vascular phenotypes similar to those of Tgfbr2 −/− , Tgfbr1 −/− and Tgfb1 −/− , namely death between 9.5 to 11.5 days post-coitum due to vascular dysgenesis, predominantly of the yolk sac but also within the embryo, in which vessels are dilated and leaky, with reduced investment of vessels by pericytes [23] , [24] , [25] , [26] . Endothelial targeting of Tgfbr1 or Tgfbr2 knockout recapitulates these vascular phenotypes [27] . Eng −/− embryos secrete reduced endothelial TGF-β1 protein levels leading to lower p-Smad2 levels in adjacent mesothelial cells, suggesting that endoglin regulates TGF-β1 production [28] . In contrast, Bmp9 −/− and Bmp10 −/− mice do not display lethal defects in yolk sac development. Bmp10 −/− mice die later in development from defective cardiac development [29] , and Bmp9 −/− animals are all viable at birth (J-K. Lee, personal communication). The situation is yet more complex since, even within a single cell, the ALK1/Smad1/5/8 and ALK5/Smad2 pathways can synergise or antagonize each other. It has been demonstrated that ALK1 directly antagonizes ALK5-mediated P-Smad2 signalling [30] . Conversely, ALK5 is required for ALK1/Smad1/5/8/ signalling in endothelial cells [30] , and phosphorylation of the cytoplasmic tail of endoglin by ALK5 can regulate ALK1/Smad1/5/8 signalling [31] . Therefore, the most likely scenario is that HHT is caused by defects in the delicate balance between endoglin, TGF-β/ALK5/ALK1 and BMP/ALK1 signalling within endothelial cells and their progenitors, with complex interactions between the various receptors and co-receptors that elicit incompletely characterized biological responses in both endothelia and adjacent pericyte cells [30] , [31] , [32] , [33] . A feature of HHT is the large intra-familial range in disease severity, suggesting that, in addition to the causative ENG or ACVRL1 mutation, independent modifier genes or environmental factors have a role in clinical severity [13] , [16] . Wounding or inflammation may be an important environmental factor precipitating development of telangiectases [34] . The notion that HHT is influenced by modifier genes is supported by the observation that a mouse model of HHT1 shows strain differences in disease severity [35] . Identification of genetic modifiers may help in development of targeted therapies. We followed the lead that different mouse strains show dramatic variation in penetrance of Tgfb1 −/− prenatal lethality [36] , [37] . Previously, we mapped genetic modifier loci, Tgfbm' s, that can suppress the lethal vascular phenotype of Tgfb1 −/− , resulting in viable, developmentally normal pups [36] , [37] , [38] . Here we demonstrate that the human PTPN14 gene, which is located in a region orthologous to mouse Tgfbm2 (ref. 37 ), shows genetic association with the presence of PAVM in HHT patients. Moreover, we show that small interfering RNA (siRNA) knockdown of endogenous PTPN14 , which encodes the protein, non-receptor tyrosine phosphatase 14 (PTPN14), modulates angiogenesis in a three-dimensional (3D) human primary endothelial culture system. PTPN14 also supports endothelial expression of EphrinB2, a key molecule required for angiogenesis [39] , establishment of endothelial arteriovenous identity [40] and recruitment of pericytes/smooth muscle cells during blood vessel wall assembly [41] . Validation of Tgfbm2 129 using C57 congenic mice Previously we showed that C57 mice that are homozygous null for the Tgfb1 tm1N allele (henceforth termed Tgfb1 −/− mice) all die prenatally from vascular dysgenesis [37] . However, on other mouse strains, namely NIH or 129, a variable fraction of Tgfb1 −/− pups are viable and developmentally normal at birth, suggesting the existence of genetic modifiers that can suppress the Tgfb1 −/− prenatal vascular phenotype [37] , [38] . By classical genetic linkage analysis of a C57 × 129 F1 intercross, we mapped a strong 129 suppressor of C57. Tgfb1 −/− pre-natal lethality to distal mouse chromosome 1, termed Tgfbm2 129 (ref. 37 ). In order to validate Tgfbm2 129 as a modifier of Tgfb1 −/− , we herein generated a C57. Tgfbm2 129/129 congenic line by backcrossing F1. C57 ×129. Tgfb1 +/− mice through >10 generations onto a C57 genetic background, using simple sequence repeat (SSR) marker-assisted breeding to select the Tgfbm2 129 allele at each generation. Homozygous C57. Tgfbm2 129/129 congenic mice harbouring 26 Mb of 129 genomic DNA around Tgfbm2 were generated and found to rescue C57. Tgfb1 −/− embryos from invariable prenatal lethality ( Fig. 1a ), providing validation for the existence of Tgfbm2 129 as a suppressor of Tgfb1 −/− embryo lethality. 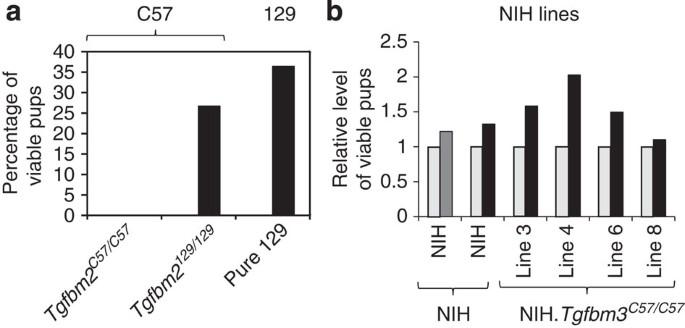Figure 1: Fine mapping and functional validation ofTgfbm2in congenic mice. (a) F1.C57/129.Tgfb1+/−mice were backcrossed >10 generations into inbred C57, at each generation selecting for both theTgfb1tm1Nallele andD1Mit362129, using genetic markers. When mice were >99.9% C57, except for a 26 Mb 129 interval at the telomeric end of chromosome 1, littermates were used to generate C57.Tgfb1+/−congenics that were either homozygous C57 (Tgfbm2C57/C57) or homozygous 129 (Tgfbm2129/129) atTgfbm2.Tgfb1+/−intercrosses within the indicated mouse strains were assayed for viableTgfb1−/−pups as a percentage of wild-type neonates. WhereasTgfb1−/−mice on a C57 (n>400) or congenic C57.Tgfbm2C57/C57(n=84) background always diein uterofrom vascular dysgenesis,Tgfbm2129/129(n=139) rescued C57.Tgfb1−/−mice from invariable prenatal lethality (P=0.02;χ2test ), almost to the extent observed on a pure 129 genetic background (n>100, and see earlier publication37). (b)Tgfb1+/−mice backcrossed >20 generations to NIH selecting only for theTgfb1tm1Nallele were unexpectedly found to harbour 129 genomic variants atTgfbm2.These mice were segregated byTgfbm2genotype and assayed for frequency of viableTgfb1−/−pups born on a NIH.Tgfbm2129/129background, compared with that on a NIH.Tgfbm2NIH/NIHbackground. A similar comparative intercross analysis was undertaken on a panel of NIH.Tgfbm3C57/C57mice (lines 3, 4, 6 and 8;n>100 mice for each genotype) that are sensitized toTgfb1−/−prenatal lethality38, showing a statistically significant association between pup viability andTgfbm2129/129(P=0.0002; logistic regression). All data in (b) are normalized relative to pup viability of the partner mouse strain homozygous for the NIH allele ofTgfbm2NIH/NIH(light grey bars). Dark grey bar shows data for NIH mice heterozygous forTgfbm2129/NIH. Black bars show data for mice homozygous 129 forTgfbm2129/129. Figure 1: Fine mapping and functional validation of Tgfbm2 in congenic mice. ( a ) F1.C57/129. Tgfb1 +/− mice were backcrossed >10 generations into inbred C57, at each generation selecting for both the Tgfb1 tm1N allele and D1Mit362 129 , using genetic markers. When mice were >99.9% C57, except for a 26 Mb 129 interval at the telomeric end of chromosome 1, littermates were used to generate C57. Tgfb1 +/− congenics that were either homozygous C57 ( Tgfbm2 C57/ C57 ) or homozygous 129 ( Tgfbm2 129/129 ) at Tgfbm2 . Tgfb1 +/− intercrosses within the indicated mouse strains were assayed for viable Tgfb1 −/− pups as a percentage of wild-type neonates. Whereas Tgfb1 −/− mice on a C57 ( n >400) or congenic C57. Tgfbm2 C57/C57 ( n =84) background always die in utero from vascular dysgenesis, Tgfbm2 129/129 ( n =139) rescued C57. Tgfb1 −/− mice from invariable prenatal lethality ( P=0.02 ; χ 2 test ), almost to the extent observed on a pure 129 genetic background ( n >100, and see earlier publication [37] ). ( b ) Tgfb1 +/− mice backcrossed >20 generations to NIH selecting only for the Tgfb1 tm1N allele were unexpectedly found to harbour 129 genomic variants at Tgfbm2. These mice were segregated by Tgfbm2 genotype and assayed for frequency of viable Tgfb1 −/− pups born on a NIH. Tgfbm2 129/129 background, compared with that on a NIH. Tgfbm2 NIH/NIH background. A similar comparative intercross analysis was undertaken on a panel of NIH. Tgfbm3 C57/C57 mice (lines 3, 4, 6 and 8; n >100 mice for each genotype) that are sensitized to Tgfb1 −/− prenatal lethality [38] , showing a statistically significant association between pup viability and Tgfbm2 129/129 ( P =0.0002; logistic regression). All data in ( b ) are normalized relative to pup viability of the partner mouse strain homozygous for the NIH allele of Tgfbm2 NIH/NIH (light grey bars). Dark grey bar shows data for NIH mice heterozygous for Tgfbm2 129/NIH . Black bars show data for mice homozygous 129 for Tgfbm2 129/129 . Full size image Co-selection of Tgfbm2 129 allele in NIH. Tgfb1 +/− mouse colony Most intriguingly, after many years of backcrossing Tgfb1 +/− mice onto another mouse strain, namely NIH/OlaHsd (NIH), and selecting only for the Tgfb1 tm1N allele at each generation (≥20 generations), we found that some NIH. Tgfb1 +/− stock mice possessed SSR markers characteristic of 129 genomic DNA on distal chromosome 1. Fine mapping delineated this 129 region to ∼ 1 Mb around D1Mit362 , that had previously been identified as the peak of Tgfbm2 by genetic linkage analysis [37] ( Supplementary Data 1 ). We designated this 1-Mb interval as the Tgfbm2 129 minimal region, and suggest that there had been biological selection for preferential inheritance of this region, driven by co-selection with the Tgfb1 tm1N allele. Fine mapping of Tgfbm2 129 in NIH congenic mice To determine whether the Tgfbm2 129 minimal region encompassed genetic variant(s) that could suppress prenatal lethality of NIH. Tgfb1 −/− embryos, we segregated NIH. Tgfb1 +/− mice according to the genotype of Tgfbm2 , that is, Tgfbm2 129/129 , Tgfbm2 129/NIH or Tgfbm2 NIH/NIH , and tested for Tgfb1 −/− prenatal loss. The viability of NIH. Tgfb1 −/− pups was enhanced somewhat by heterozygosity for Tgfbm2 129/NIH , and to a greater extent by homozygosity at Tgfbm2 129/129 ( Fig. 1b ). However, due to the already high developmental viability of Tgfb1 −/− mice when on a NIH background, this increase was not statistically significant. We therefore sensitized the NIH mice to Tgfb1 −/− prenatal loss by breeding in another modifier locus, Tgfbm3 C57 , that we previously reported to accentuate Tgfb1 −/− prenatal loss [38] . Sensitized NIH. Tgfbm3 C57/C57 congenic lines, 3, 4, 6 and 8 ( Fig. 1b ), which each harbour different intervals of C57 genomic DNA at Tgfbm3 (K.K.K. and R.J.A. unpublished observations), were bred into NIH. Tgfbm2 129/129 mice. These were intercrossed to re-generate homozygosity at NIH. Tgfbm3 C57/C57 and segregated by Tgfbm2 genotype into either Tgfbm2 129/129 or Tgfbm2 NIH/NIH . Importantly, homozygosity for Tgfbm2 129/129 suppressed Tgfb1 −/− prenatal lethality in every line, showing statistical significance when assessed by logistic regression analysis ( Fig. 1b ; odds ratio=2.03; confidence interval=1.41–3.03, P= 0.0002; logistic regression). The 1-Mb Tgfbm2 129 minimal interval therefore harbours a Tgfb1 −/− suppressor effect, giving credence to the notion that inheritance of Tgfbm2 129 on the NIH background was driven by biological co-selection with the Tgfb1 tm1N allele. Fine genetic mapping by SSR, single nucleotide polymorphism (SNP) and sequence analysis refined the map location of the Tgfbm2 minimal region and excluded the nearby Tgfb2 gene ( Fig. 2a ), which might otherwise be considered an obvious candidate to modify Tgfb1 function. 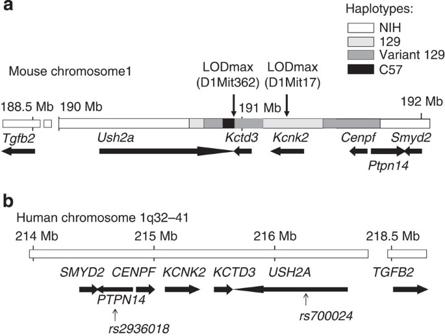Figure 2: Genomic structure of murineTgfbm2and humanTGFBM2. (a) The murineTgfbm2locus, indicating the position of the co-selected 1-MbTgfbm2129minimal interval (boxed region) spanning from exons 57–60 ofUsh2ato exons 2–6 ofPtpn14. Also indicated are 129S2Sv, C57 and 'variant 129' haplotypes within this minimalTgfbm2interval, together with the positions of the peak genetic linkage from the original genetic mapping of this locus37. (b) Human 1q41 region syntenic toTgfbm2, indicating position ofPTPN14SNPrs2936018andUSH2ASNPrs700024. Figure 2: Genomic structure of murine Tgfbm2 and human TGFBM2 . ( a ) The murine Tgfbm2 locus, indicating the position of the co-selected 1-Mb Tgfbm2 129 minimal interval (boxed region) spanning from exons 57–60 of Ush2a to exons 2–6 of Ptpn14 . Also indicated are 129S2Sv, C57 and 'variant 129' haplotypes within this minimal Tgfbm2 interval, together with the positions of the peak genetic linkage from the original genetic mapping of this locus [37] . ( b ) Human 1q41 region syntenic to Tgfbm2 , indicating position of PTPN14 SNP rs2936018 and USH2A SNP rs700024. Full size image Fine mapping analysis across the minimal Tgfbm2 129 region revealed two major haplotype blocks that were identical to 129S2SV/Hsd, the 129 sub-strain used in our laboratory. However, there were also two additional haplotype blocks distinct from 129S2SV/Hsd, despite the fact that they share more similarity to 129S2SV/Hsd than either C57 or NIH. We termed these haplotypes 'variant 129' in Fig. 2a and Supplementary Data 1 . Their existence suggests that the Tgfbm2 129 minimal DNA may have derived from another 129 sub-strain that had been bred into the colony earlier during the propagation of the Tgfb1 tm1N allele [42] . TGFBM2 associates with the presence of PAVM in Dutch HHT As homozygous mouse gene knockouts of the causative genes for HHT, Eng and Acvrl1 , phenocopy the vascular dysgenesis seen in Tgfb1 −/− embryos [25] , [26] , [40] , and because Tgfbm2 suppresses this phenotype ( Fig. 1a,b ), we investigated SNPs within human orthologues of the Tgfbm2 genes for genetic association to HHT clinical severity. We initially investigated 721 individuals from 137 different families who had been molecularly screened for the causative HHT mutation and clinically screened for the presence of PAVMs as a parameter of severity [13] . The human genome at 1q41 shows synteny with mouse over the Tgfbm2 minimal region ( Fig. 2b ), and gene-centric tag-SNPs ( n =76) covering the five orthologous Tgfbm2 genes were selected, together with tag-SNPs ( n =15) covering SMYD2 and TGFB2 , which are located 20 Kb proximal and 1.9 Mb distal to TGFBM2 , respectively ( Fig. 2b ). Additionally, 443 tag-SNPs were included that covered 72 'candidate genes' selected on the basis of involvement in TGF-β signalling or responses, and located all around the genome ( Supplementary Data 2 ). The first screen included 649 Dutch individuals of northern European descent and 72 Afro–Caribbean individuals from the Dutch Antilles ( Table 1 and Supplementary Table S1 ). We used a modification of the transmission disequilibrium test (TDT), namely Gamete Competition (GC) [43] , to screen for genetic association with the presence versus absence of PAVM in HHT mutation carriers. GC was selected over TDT because of the large, multigenerational structure of families within this cohort ( Supplementary Table S2 and S3 ). A total of 29 of the 534 SNPs screened showed nominal evidence of over-transmission to PAVM+ HHT patients ( P <0.05, GC test) ( Fig. 3a ) and were genotyped in an additional 108 northern European Dutch individuals. Although this smaller data set was not significant alone, when pooled with the first data set, 4 of the 29 SNPs showed improvements in P -value in excess of one order of magnitude, all were within TGFBM2 , three within the gene PTPN14 ( rs2936018, P =3×10 −5 ; rs2936017 , P =2×10 −4 ; rs3002300 , P =2×10 −4 ; GC test) and one 1.7 Mb distal to PTPN14 , within USH2A ( rs700024, P =1.6×10 −3 ; GC test) ( Fig. 3b , Table 2 ). Table 1 Number of individuals and families in the Dutch screen. 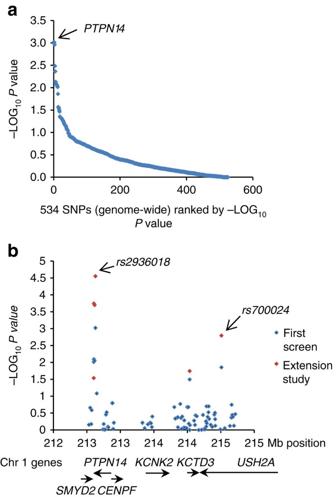Figure 3: SNPs withinPTPN14show genetic association with presence of PAVM in Dutch HHT patients. (a) A total of 534 gene-centric SNPs tagging the five syntenic genes ofTGFBM2at 1q41,plus 72 TGFβ/BMP signalling 'candidate genes', were screened in 721 HHT patients and family members. Graph shows the distribution of–log10(P)values resulting from GC analysis of genetic association to PAVM in pooled HHT1 and HHT2. (b) The genomic map distribution of–log10(P)values at 1q41 for 76 gene-tagging SNPs across theTGFBM2across. Black data points represent initial Dutch SNP screen; Red data points represent cumulative–log10(P)values for combined initial and extension studies of Dutch patient samples. Full size table Figure 3: SNPs within PTPN14 show genetic association with presence of PAVM in Dutch HHT patients. ( a ) A total of 534 gene-centric SNPs tagging the five syntenic genes of TGFBM2 at 1q41,plus 72 TGFβ/BMP signalling 'candidate genes', were screened in 721 HHT patients and family members. Graph shows the distribution of –log 10 (P) values resulting from GC analysis of genetic association to PAVM in pooled HHT1 and HHT2. ( b ) The genomic map distribution of –log 10 (P) values at 1q41 for 76 gene-tagging SNPs across the TGFBM2 across. Black data points represent initial Dutch SNP screen; Red data points represent cumulative –log 10 (P) values for combined initial and extension studies of Dutch patient samples. Full size image Table 2 Gamete Competition output values in initial Dutch screen (IS) and IS pooled with the extension study (IS + EXT). Full size table To validate the GC result, we broke up large HHT family structures into nuclear families and ran TDT in 19 informative family trios. Both rs2936018 and rs2936017 within PTPN14 showed significant over-transmission of the minor allele to PAVM+ HHT individuals ( P =8×10 −3 ; TDT). Only one other SNP, rs700024 , was similarly found to be associated with PAVM by TDT ( P =9×10 −3 ; TDT) ( Figs 2b , 3b ). PTPN14 genetic association in both Dutch HHT1 and HHT2 To further validate the genetic association to PAVM, we analysed the Dutch HHT1 and HHT2 families independently. rs2936017 and rs2936018 , located within PTPN14 , were the only SNPs to show nominal evidence of over-transmission to PAVM+ in both HHT1 ( P =0.01 and P <0.01, respectively, GC test, Table 2 ) and HHT2 ( P <0.01 and P =0.001, respectively, GC test, Table 2 ), demonstrating replication of genetic association in two unrelated HHT patient populations, with causative mutations in two different genes. PTPN14 genetic association is not due to linked TGFB2 gene PTPN14 SNP rs2936018 ( P =3×10 −5 ) and USH2A SNP rs700024 ( P =1.6×10 −3 ) are 2.8 MB and 1.9 Mb, respectively, from the 5′ end of the TGFB2 gene ( Fig. 2b ). As variant TGFB2 is a logical biological candidate for modulating TGF-β1 action and, as one SNP in TGFB2 (rs1891467 ) showed nominal evidence of association with PAVM in the preliminary HHT screen ( P =5.5×10 −3 ; Table 2 ), we tested linkage disequilibrium (LD) between TGFB2 and the rs700024 haplotype block. We also tested whether families that contributed to the nominal TGFB2 association were the same as those contributing to the USH2A and PTPN14 associations. There was no LD between these haplotype blocks ( r 2 <0.2). Moreover, the families contributing most strongly to TGFB2 association were different from those contributing to association with PTPN14 or USH2A , suggesting that genetic association with rs2936017, rs2936018 or rs700024 is not driven by genetic linkage to TGFB2 . PTPN14 association to PAVM validated in French HHT2 The 29 nominally associated SNPs from the initial Dutch screen were subsequently genotyped in an independent French replication cohort of 222 individuals, all with HHT (mostly HHT2; n =146) and screened for PAVM [16] . The relatively small number of HHT1 patients in the French population ( n =76) prevented an independent analysis of genetic association in this specific monogenic disorder. However, the French HHT2 population was sufficiently large for independent analysis. Of the 29 SNPs tested, only 3 SNPs showed nominal evidence of genetic association to PAVM+ in French HHT2 ( P <0.05, GC test), precisely those PTPN14 SNPs most strongly associated in Dutch HHT1 and HHT2 ( Table 3 ). Table 3 Gamete Competition results across TGFBM2 in French HHT. Full size table siPTPN14 enhances angiogenesis in 3D EC culture Very little is known about the action of PTPN14 in vascular endothelial cells, although this protein is expressed at high levels in human umbilical vein endothelial cells [44] , as well as human umbilical artery endothelial cells (HUAECs) and HMEC-1 microvascular endothelial cells ( Fig. 4a ). The strong genetic association of PTPN14 with PAVM in HHT led us to investigate a possible function for this protein in endothelial cell biology. As HHT has been suggested to be a disease of excessive angiogenesis [45] , [46] , [47] , we chose to use an in vitro angiogenesis assay. We first optimized knockdown of PTPN14 protein levels using siPTPN14 ( Fig. 4a ). Then, without a preconceived model as to the mode of action of the causative PTPN14 genetic variant(s), we investigated the effect of siRNA knockdown of PTPN14 in a 3D in vitro angiogenesis assay ( Fig. 4b ). Interestingly, siPTPN14 moderately, but significantly, enhanced angiogenic sprouting of primary HUAECs, as well as significantly increasing the numbers of endothelial tip cells ( Fig. 4b,c ), giving credence to the notion that PTPN14 is innately involved in the regulation of endothelial angiogenesis, as least in this in vitro system. 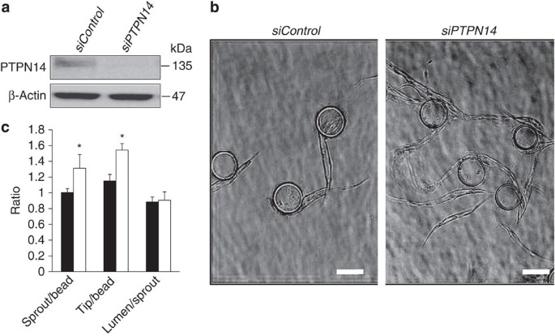Figure 4:siPTPN14stimulatesin vitroangiogenesis. si-RNA KD ofPTPN14was optimized in HMEC-1 cells (a) and HUAECs (not shown) by western analysis. (b,c) siRNA-treated HUAECs were cultured for 6 days in a 3Din vitroangiogenesis assay. (b) Phase contrast micrographs ofsiControlorsiPTPN14-treated HUAEC at 6 days. Scale bar represents 150 μm. (c) Vascular sprouts longer than one bead diameter (150 μm), sprouts with and without lumens, and tip cells were enumerated by morphology under phase contrast microsopy. Tip cell number is a surrogate for branching, and lumen formation is a parameter of advanced angiogenesis. Graph shows quantification of the ratios of sprouts per bead, tip cells per bead and lumens per sprout, after treatment withsiControl(black) orsiPTPN14(white). The analysis was performed blinded to sample identity. At least 25 beads in three different wells were analysed for each experiment. Two biological replicates were undertaken. Results from one representative experiment are shown. Mean and s.d. are shown. *P<0.01, Studentst-test. Figure 4: siPTPN14 stimulates in vitro angiogenesis. si-RNA KD of PTPN14 was optimized in HMEC-1 cells ( a ) and HUAECs (not shown) by western analysis. ( b , c ) siRNA-treated HUAECs were cultured for 6 days in a 3D in vitro angiogenesis assay. ( b ) Phase contrast micrographs of siControl or siPTPN14 -treated HUAEC at 6 days. Scale bar represents 150 μm. ( c ) Vascular sprouts longer than one bead diameter (150 μm), sprouts with and without lumens, and tip cells were enumerated by morphology under phase contrast microsopy. Tip cell number is a surrogate for branching, and lumen formation is a parameter of advanced angiogenesis. Graph shows quantification of the ratios of sprouts per bead, tip cells per bead and lumens per sprout, after treatment with siControl (black) or siPTPN14 (white). The analysis was performed blinded to sample identity. At least 25 beads in three different wells were analysed for each experiment. Two biological replicates were undertaken. Results from one representative experiment are shown. Mean and s.d. are shown. * P <0.01, Students t -test. Full size image ALK1 and EphrinB2 show interdependent expression with PTPN14 It has been suggested that HHT pathology might be attributed to excess angiogenesis, as some patients respond favourably to treatment with the VEGF inhibitor, bevacizumab [45] , [46] , and to the angiogenesis inhibitor, thalidomide [47] . A defect in specification of arteriovenous identity has also been implicated as both Eng −/− and Acvrl1 −/− embryos show loss of arterial identity at the expense of expansion of venous vessels [40] , [48] , [49] . Moreover, Acvrl1 −/− embryos fail to upregulate Efnb2 , which encodes EphrinB2, a guidance molecule known to be pivotal in tip cell-mediated angiogenesis [50] , [51] and best known as a marker and effector of arterial versus venous endothelial cell specification [39] , [50] , [51] . This dependence of EFNB2/ EphrinB2 expression on ACVRL1 has also been observed in cultured HUAECs (J-H.K, M.R.P., S.C.G. and C.C.W.H. unpublished observations) ( Fig. 5a,b ). Interestingly, we found that siPTPN14 knockdown in cultured HUAECs also resulted in a dramatic reduction in EFNB2/ EphrinB2 expression at both RNA ( Fig. 5c ) and protein levels ( Fig. 5d ). Conversely, knockdown of EFNB2 or ACVRL1 significantly elevated PTPN14 gene expression ( Fig. 5e ) and protein levels ( Fig. 5f ), demonstrating interdependence for expression between these three genes ( Fig. 5g ). Thus, PTPN14 may interact with ACVRL1 and EFNB2 , directly or indirectly, to regulate angiogenesis and/or arteriovenous specification, both processes that are implicated as abnormal in the pathology of HHT [40] , [45] , [48] , [52] . 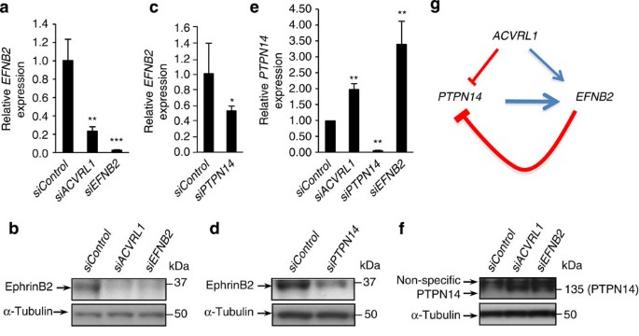Figure 5:ACVRL1andEFNB2show interdependent expression withPTPN14 in vitro.(a–f) HUAECs were treated with indicated siRNAs, and cultured for 2 days. Quantitative reverse transcription–PCR (a,c,e) and western blot analysis (b,d,f) were then performed forEFNB2/EphrinB2 (a–d) andPTPN14(e,f). (g) Cartoon summary of possible interactions implied by data in (a–f);PTPN14downregulation byACVRL1may be directly or indirectly mediated via elevatedEFNB2levels. Data in panelsa, candeare representative of at least three independent biological replicates. Data in panelsb, dandfare representative of two independent biological replicates. Moreover, data in panelsb, dandfare from additional experiments, independent from those shown ina, cande. Mean and s.d. are shown. ***P<0.0001, **P<0.001, *P<0.01, Studentst-test. Figure 5: ACVRL1 and EFNB2 show interdependent expression with PTPN14 in vitro. ( a–f ) HUAECs were treated with indicated siRNAs, and cultured for 2 days. Quantitative reverse transcription–PCR ( a,c,e ) and western blot analysis ( b,d,f ) were then performed for EFNB2/ EphrinB2 ( a–d ) and PTPN14 ( e,f ). ( g ) Cartoon summary of possible interactions implied by data in ( a–f ); PTPN14 downregulation by ACVRL1 may be directly or indirectly mediated via elevated EFNB2 levels. Data in panels a, c and e are representative of at least three independent biological replicates. Data in panels b, d and f are representative of two independent biological replicates. Moreover, data in panels b, d and f are from additional experiments, independent from those shown in a, c and e . Mean and s.d. are shown. *** P <0.0001, ** P <0.001, * P <0.01, Students t -test. Full size image Here, we validated the action of Tgfbm2 129 as a suppressor of prenatal vascular lethality of Tgfb1 −/− mice on two different genetic backgrounds, NIH and C57. Intriguingly, we discovered a 1-Mb interval of 129-like genomic DNA spanning the Tgfbm2 locus in our NIH. Tgfb1 +/− mouse stock that had unintentionally been selected in our breeding protocol. The ability of this minimal Tgfbm2 129 interval to suppress the lethal vascular dysplasia of Tgfb1 −/− embryos suggests that this genomic element had been selectively inherited through multiple generations, driven by co-selection with the Tgfb1 tm1N allele. Interestingly, although the minimal Tgfbm2 129 interval shared two extensive haplotype blocks with the 129 sub-strain that we have used in our lab for many years, around half of the 1-Mb interval was genetically distinct from all mouse lines in our animal unit. It is therefore probable that this minimal Tgfbm2 129 region derived from a related 129 sub-strain onto which the Tgfb1 tm1N allele was initially bred [42] before our genetic studies. This minimal Tgfbm2 129 interval might even lead back to the 129 embryonic stem cells on which the original Tgfb1 tm1N allele was generated [42] , although we have been unable to validate this thesis. Suppressor screens utilizing sensitized genetic stock have for years been used in lower organisms, such as Drosophila and Caenorhabditis elegans , to identify genes that interact on specific signalling pathways. Our current report is the first evidence of such a mechanism occurring naturally in mice without experimental mutagenesis. Importantly, hundreds of genetically engineered mouse models are now available. Many have been bred into different inbred genetic backgrounds over several years. Genome-wide screens for unlinked genetic variants that are co-inherited with a recombinant genetic locus could be generally applied to identify novel genes and mechanisms involved in signalling and developmental pathways in vivo , as well as genetic interactions that contribute to human disease susceptibility. In a previous study, it was shown that breeding the Eng +/− mouse onto a 129/Ola genetic background potentiated the appearance of vascular lesions in adult mice, whereas the C57 strain was resistant [35] . This might appear incongruent with our observation of suppression of Tgfb1 −/− embryo lethality by the 129 allele of Tgfbm2 , but there are several possible explanations for this discrepancy. First, 129/Ola is distinct from the 129 sub-strain used in the current study. Second, genetic modifier interactions are complex and, within an individual mouse strain, different modifier loci may have negative or positive effects on the trait in question. Furthermore, distinct modifiers can have synergistic or antagonistic effects on each other. Nevertheless, the identification of natural genetic variants that have such profound effects on in vivo pathology provides insight into the molecular mechanisms of disease. Most importantly, we showed that PTPN14 within the orthologous human TGFBM2 locus showed the strongest genetic association to PAVM in HHT. This was despite screening over 500 SNPs, >450 of which informed on 72 other genes selected as candidate modifiers on the basis of being components of the TGF-β and BMP signalling or response pathways. Genetic association of PTPN14 to PAVM was then validated in two independent HHT diseases, HHT1 and HHT2, and in two independent populations, Dutch and French HHT, providing robust evidence that variants in this gene alter risk for PAVM in HHT patients. This finding is of significant clinical relevance in elucidating the molecular pathology of PAVM. We then demonstrated that knockdown of the endogenous PTPN14 gene in cultures of primary human endothelial cells modulates angiogenesis in a 3D culture assay and alters the expression of EphrinB2, a well characterized regulator of angiogenesis [50] , [51] and arteriovenous specification [39] , suggesting an involvement of PTPN14 in these processes, and lending further support to the notion that HHT is a disease of angiogenesis and arteriovenous specification. The route from a genetic modifier of Tgfb1 −/− phenotype to identification of a genetic risk factor for PAVM in HHT provides support to the notion of TGF-β1 involvement in the pathology of PAVM in HHT, whether primary or secondary. It does not, however, rule out a role for BMP9 and BMP10, but is supportive of an imbalance in signalling between these two TGF-β superfamily pathways. Little is known about non-receptor tyrosine phosphatase 14 (PTPN14) function. It is expressed at high levels in endothelial cells [44] , and it was recently found to be mutated in a single family with a rare case of recessive human lymphedema-choanal atresia syndrome [53] . Preliminary studies have suggested a direct interaction between PTPN14 and VEGF-R3 that regulates signalling from VEGF-C [53] . As VEGF-R3 has been shown to be important in angiogenesis [54] , as well as lymphangiogenesis, this would support a role for PTPN14 in determining HHT disease severity. Nevertheless, there is still much to be investigated concerning the mechanisms of action of PTPN14, and there are seemingly contradictory reports on its function in the literature. This protein has alternatively been reported as an inactive phosphatase [55] or as actively involved in dephosphorylation of β-catenin [56] . It has also been shown to both stabilize and destabilize adherens junctions [56] , [57] , and to affect TGFβ1 secretion [57] . The possession of a FERM domain and potential SH3 domain may suggest a role for PTPN14 as an adaptor protein in signal transduction. Future studies will include analysis of the protein partners that interact physically with PTPN14 not only in endothelial cells, but also in pericytes and smooth muscle cells, which are secondarily impacted in HHT pathology. Further analysis of the nature and differential activity of human PTPN14 variants would be informative as to protein function and altered molecular interactions that may suggest novel routes to medical intervention. In conclusion, the identification of PTPN14 as a genetic modifier of PAVM in HHT provides novel insight into the molecular circuitry operating in vascular cells of HHT patients. This finding will contribute to an understanding of the molecular mechanisms underlying PAVM formation that might ultimately be used in drug development for HHT or other disorders of angiogenesis. Mouse studies All animal experiments were undertaken at UCSF, and were in full compliance with the UCSF Institutional Animal Care and Use Committee (Protocol AN085727), which is AAALAC accredited. Mice were housed in a SPF facility in individually ventilated microisolator caging with paper chip bedding and unlimited access to lab diet irradiated feed (Lab Products™) and water. Housing temperature was maintained between 20 and 22 °C, and lighting adjusted to a 12-h light–dark cycle with 30–70% humidity. Mice were handled only in sterile BSL2 laminar flow hoods. They were housed as breeding trios (1♂ , 2♀) until pups were 3 weeks of age, and then at a maximum of five same sex animals per cage. Both genders of animal were used for study, and no sex differences were observed. The Tgfb1 tm1N allele (also termed Tgfb1 -) [42] was bred onto three different genetic backgrounds by repeated backcross (>10 generations) to inbred C57BL/6NTac (C57), NIH/OlaHsd (NIH) or 129S2/SvHsd (129). Human subjects Dutch Caucasians and Dutch Antillean Blacks were selected from a panel consisting of probands and family members screened for HHT. All manifestations of HHT were recorded for both probands and family members. The clinical diagnosis of HHT was established according to the Curaçao criteria [7] , [8] , which are clinical features of epistaxis, multiple telangiectases, visceral AVM and a first-degree relative with HHT. A diagnosis of HHT is considered definitive if three criteria are present, possible if two criteria are present and unlikely if fewer than two criteria are present. Mutation carrier status was confirmed by molecular analysis. Most probands and family members were screened for visceral manifestations at St Antonius Hospital, which specializes in the diagnosis and treatment of HHT. In most cases, screening for the presence of a PAVM was performed routinely by chest radiography and by measuring partial oxygen tension in arterial blood and, if abnormal, followed by the 100% oxygen right-to-left shunt test. Patients with a suspected PAVM were offered conventional angiography, digital subtraction angiography of the pulmonary arteries or computed tomography (CT) of the chest. In some patients, PAVMs were diagnosed using high-resolution CT and/or contrast trans-thoracic echocardiography. French HHT clinical diagnosis was also established according to the Curaçao criteria [17] . Mutation carrier status was confirmed by molecular diagnosis (heteroduplex analysis or denaturing high performance liquid chromotography and sequencing). Screening for PAVMs was recommended to asymptomatic patients and accepted by a majority of them (66.8%) [16] . The diagnosis of pulmonary involvement was made either in patients presenting symptoms (for example, dyspnoea and cyanosis) or complications (mainly brain abscess), or in asymptomatic HHT patients who underwent screening using contrast trans-thoracic echocardiography, chest radiograph and/or oxygen shunt test as described. The 222 French patients included in the present study all carried a mutation in either ENG or ACVRL1 , and 43% of them had a PAVM (74% for HHT1 patients and 27% for HHT2 patients). Familial structures included 111 singletons, 40 duos, 2 trios, 5 quartets and 1 family with 5 individuals. Study protocols were approved by local ethics committees at all institutions, and informed consent was obtained from each subject before participation in the studies. Human SNP selection Gene-centric tag-SNPs within and flanking TGFBM2 at 1q41, and within and flanking candidate genes, were utilized. SNPs were chosen on the basis of being non-synonymous coding polymorphisms, potential splice site variants or inferred to disrupt important gene regulatory sites (that is, microRNAs and transcription factor binding sites, and so on) using the UCSC genome server. We further looked for SNPs located in highly conserved regions in the 3′ UTR. This first set of SNPs was complemented by tag-SNPs using a tag approach with the HapMap phase II database ( http://www.hapmap.org ) by 'force including' the first set of variants using the Haploview Tagger and by searching for additional tag-SNPs. Selected SNPs were estimated to give ∼ 85% coverage of any chosen gene. Human genotyping and quality control Initial genotyping of the Dutch cohort was performed using 750-ng labelled genomic DNA hybridized to a custom Illumina chip. Genotyping for the extension and replication studies, and for fine mapping, was performed using Sequenom MALDI-TOF mass spectrometry. No significant difference in call rates between cases and controls was seen. Samples successfully genotyped in <95% of markers were excluded from analysis. Markers were excluded if they deviated significantly from Hardy–Weinberg equilibrium ( P <0.05, Hardy–Weinberg) or if they had a call rate <95% in the entire cohort. In vitro angiogenesis assay The in vitro model was performed as described previously [58] . Briefly, primary human umbilical artery endothelial cells (HUAECs) from Lonza were coated onto Cytodex3 beads (Sigma-Aldrich Co., 200 cells per bead, 250 beads per well) and cultured in fibrin gels in EGM2 medium (Invitrogen). Normal human lung fibroblasts were plated on top of the gel. After 6–8 days, beads were photographed and the sprouts whose lengths were greater than the diameter of the bead were counted under an Olympus IX70 inverted phase contrast microscope. At least three wells were assayed for each sample, and a minimum of 25 beads per well were counted. Before coating onto beads, the ECs were loaded with siRNA (13 pmole per 6-well plate) using Lipofectamine 2000 (Invitrogen). siRNA transient transfection and analysis ON-TARGETplus SMARTpool siRNA oligonucleotides specific for PTPN14 were obtained from Dharmacon (J-008509-05, 5′-GAAGACAAGCGGUAAUAUA-3′; J-008509, 5′-CATAACAAGUCGACCAUUC-3′; J-008509-07, 5′-GCUAAUGAGCCUUUGCUUU-3′; J-008509-08, 5′-GGUGAGCACUACUCGGAAA-3′). ACVRL1 (5′-GGAUCAAGAAGACACUACATT-3′) and EFNB2 (5′-GACAAGGACUGGUACUAUATT-3′) siRNAs were obtained from Ambion. HUAECs, grown in M199 media (Invitrogen), were transiently transfected with each siRNA (13 pmole per 6-well plate) or their corresponding scrambled siRNA controls using Lipofectamine 2000 (Invitrogen). At 48 h after transfection, gene and protein expression were analysed by quantitative reverse transcription–PCR and/or western blot. Quantitative reverse transcription–PCR Total RNA was isolated from the cells with RNeasy Plus Mini Kit (Qiagen). 1 μg RNA was used for first strand cDNA synthesis with iScript cDNA Synthesis kit (Bio-Rad). Primer sequences for EFNB2 (GenBank accession number, NM_004093 ) were 5′-TTCGACAACAAGTCCCTTTG-3′ (sense) and 5′-GATGTTGTTCCCCGAATGTC-3′ (antisense); for ACVRL1 (GenBank accession number, NM_000020 ) were 5′-TTGGGCACCACATCATAGAA-3′ (sense) and 5′-GACTGACATCTGGGCCTTTG-3′ (antisense); for PTPN14 (GenBank accession number, NM_005401 ) were 5′-CAGGGAGTGAATGTGATTC-3′ (sense) and 5′-CAGTATCGGTGGCTTTTGGT-3′ (antisense) and for GAPDH (GenBank accession number, NM_002046.3 ) were 5′-AATCCCATCACCATCTTCCA-3′ (sense) and 5′-TGGACTCCACGACGTACTCA-3′ (antisense). All primer pairs crossed intron–exon boundaries, thereby avoiding background contamination from genomic DNA. PCR was performed using an IQ5 real time PCR system (Bio-Rad) with SYBR green quantification. Gene expression was normalized to GAPDH expression levels. Western blot analysis Cells were lysed on tissue culture plates using ice-cold RIPA buffer (50-mM Tris–HCL, pH 7.4, 150-mM sodium chloride, 1% NP40 and 0.1% SDS) supplemented with protease inhibitor cocktail tablets (Roche). Samples were run on 4–12 or 3–8% SDS–PAGE and transferred to an Immobilon-P PVDF membrane (Millipore). Western blots were probed overnight at 4°C with rabbit anti-PTPN14 1:1,000 (Abcam), rabbit anti-EphrinB2 1:1,000 (Abcam), rabbit anti-α-tubulin 1:10,000 (Sigma) or HRP-conjugated anti-β-actin 1:10,000 (Cell Signaling) primary antibodies. The secondary antibody used was HRP-conjugated anti-rabbit antibody (GE healthcare). Mouse genetics Comparison of percentage Tgfb1 −/− pup viability was undertaken by χ 2 analysis ( Fig. 1a ). In Fig. 1b , for comparisons across multiple strains, we fit a logistic regression model with birth status as the responsive variable and mouse line as the independent variable, and performed the likelihood ratio test of this model over the model with only the mouse line as the effect. For analysis within each line, we fit a logistic regression model with birth status as the response variable and strain as the independent variable, and performed the likelihood ratio test of this model over the null model. Human family-based analysis Statistical power was determined using the Quanto program ( http://hydra.usc.edu/gxe ). Familial association analyses were carried out using the GC model implemented in the software package MENDEL [43] . The GC model is an application of the Bradley–Terry method of ranking, which compares the observed number of transmissions of the at-risk allele from heterozygous parent to affected offspring, to the expected transmissions (50%) [43] , [59] . The best associations were validated using the Family Based Association Testing (FBAT) program, which correlates genotypes, conditional on parents, with the phenotypes. The FBAT analyses were carried out both with and without unaffected individuals. The GC included the unaffected individuals as the model uses full pedigree data. Multiple testing issues in the family-based analyses were addressed using the false discovery rate method and SNP spectral decomposition [60] and permutation analysis that take into consideration the inter-SNPs correlations. We performed 1,000 permutations for each family-based analysis. The SNP spectral decomposition and permutation analysis gave similar cutoff of significance. How to cite this article: Benzinou, M. et al . Mouse and human strategies identify PTPN14 as a modifier of angiogenesis and hereditary haemorrhagic telangiectasia. Nat. Commun. 3:616 doi:10.1038/ncomms1633 (2012).